Repeated evolution in overlapping mimicry rings among North American velvet ants Müllerian mimicry, in which two or more harmful species share a similar appearance for mutual benefit, is a widely appreciated, yet relatively uncommon natural phenomenon. Although Müllerian mimicry occurs in vertebrates, most studies are focused on tropical, herbivorous invertebrates. Here we identify a large Müllerian mimicry complex in North American velvet ants (Hymenoptera: Mutillidae). These are conspicuous, diurnal parasitoids of bees and wasps that defend themselves with a powerful sting. We investigate morphological and genetic variation and ask whether morphological similarities are the result of convergent evolution or shared ancestry. We find that 65 species in the velvet ant genus Dasymutilla can be placed into one of six morphologically distinct and geographically delimited mimicry rings. Müllerian colour patterns are primarily the result of independent evolution rather than shared, phylogenetic history. These convergent colour syndromes represent one of the largest known Müllerian mimicry complexes yet identified, particularly in the Northern Hemisphere. Müllerian mimicry, a mutualism in which two or more species with effective secondary defenses share a similar appearance for mutual benefit [1] , is a well-known, yet relatively uncommon natural phenomenon. Although Müllerian mimicry rings—groups of species that benefit from shared aposematic signals—have been documented from a variety of taxa, including reptiles, amphibians and arthropods (reviewed by Ruxton et al . [2] ), the most well-known examples are lepidopteran (butterflies and moths) (for example, refs 3 , 4 ), with the Neotropical butterfly genus Heliconius among the most celebrated model systems [5] . Although Müllerian mimicry has been recognized in some Nearctic species [6] , species-rich mimicry rings are more often documented in tropical taxa. The apparent higher incidence of mimicry in the tropics has led to the postulation that mimicry might evolve more easily at lower latitudes due to higher predator and prey diversities [7] , but more studies on non-lepidopteran groups [2] and from non-tropical taxa are needed to better understand this phenomenon. Velvet ants, which are actually wingless wasps (Hymenoptera: Mutillidae), are a common, yet often overlooked, component of many North American habitats and are becoming a model system for historical biogeography in North American deserts [8] , [9] . Among velvet ants, the females of the diurnal genus Dasymutilla are aposematically coloured and are protected by a suite of secondary defenses, which often include stridulation (auditory aposematism), pungent exudate secretions, a hard cuticle and a painful sting [10] . Although velvet ants primarily parasitize the nests of potentially dangerous hosts (solitary bees and wasps), their well-defended nature likely evolved in response to predation pressures [10] , [11] , [12] . Velvet ants are diverse and abundant in xeric habitats and are active at the same time as most diurnal terrestrial lizards, yet analyses of gut contents show that most insectivorous lizards rarely feed on velvet ants [11] . Feeding trials have revealed that lizards will consume slender, ant-like velvet ants, but most lizards either avoid the aposematically coloured species [10] , [11] , [12] , or quickly learn to recognize and avoid them [11] , [13] . The latter result, that lizards learn to recognize and avoid aposematic velvet ants, indicates that the colour patterns are effective in defence and in training potential predators. The effectiveness of velvet ant defenses has likely been influential in the evolution of various Batesian mimics, harmless species imitating the warning signals of harmful species [14] . Known Batesian mimics of velvet ants include various beetles [15] , [16] , [17] , spiders [18] , [19] and antlion larvae [20] . In addition to other taxa mimicking velvet ants, several authors have noted the phenotypic similarity among unrelated velvet ant species, but only within a taxonomic context [21] , [22] , [23] . The possibility of velvet ant Müllerian mimicry rings, however, has not been suggested, yet a few species are thought to mimic true ants [10] , [24] . Here we report on one of the largest Müllerian mimicry complexes yet to be identified, with at least 65 North American Dasymutilla species involved in six distinct mimicry rings. While structural morphological characters can often be used to distinguish each of these species, multiple geographically concordant colour forms are present within and among species. In other groups, including birds and butterflies, analyses have found that some of the similarities in supposed mimetic traits can be best explained by phylogenetic relatedness rather than through repeated or independent evolutionary events [6] , [25] , [26] . The goals of this paper are twofold: first, to describe morphological variation among female Dasymutilla velvet ants that potentially comprise multiple, overlapping mimicry rings; and second, to investigate the phylogenetic context in which mimetic phenotypes have evolved. The latter objective allows us to determine if morphologies involved in Müllerian mimicry have evolved multiple times, or if different phenotypes represent single evolutionary origins. Description of mimicry complex Velvet ants in the genus Dasymutilla are widespread in the New World, ranging from Peru to Canada. We examined mimetic patterns in the females of 65 Dasymutilla species ( Supplementary Table S1 ) from across North America and found that six common colour forms are present, representing six geographically based mimicry rings ( Fig. 1 ). In addition to the 65 species treated here, most of the remaining 46 recognized Dasymutilla species (out of a total of 113 North American species known from females) can also reliably be assigned to one or more of these mimicry rings but will not be included in the following description of mimicry rings because of the lack of available molecular data from these species. This species-rich Müllerian mimicry complex, therefore, potentially represents one of the largest known mimicry complexes worldwide. These Dasymutilla mimicry rings are based on shared colour patterns and geographic location. We used non-metric multidimensional scaling (NMDS) and a permutational multivariate analysis of variance (PERMANOVA) to quantify and examine the morphological similarity and differences among species in each putative mimicry ring using seven colour characters and one setal character (see Methods for description of characters). Although the PERMANOVA does not account for phylogenetic non-independence, this was tested using other analyses (see the ‘Phylogenetic reconstructions’ section below). These analyses, NMDS and PERMANOVA, indicated that each of the six mimicry rings is morphologically distinct: the overall effect of mimicry ring as a categorical variable was F =34.175, R 2 =0.737, P <0.001; furthermore, pairwise analyses supported the morphological distinctness of each of the rings ( Supplementary Table S2 , Fig. 2 ). 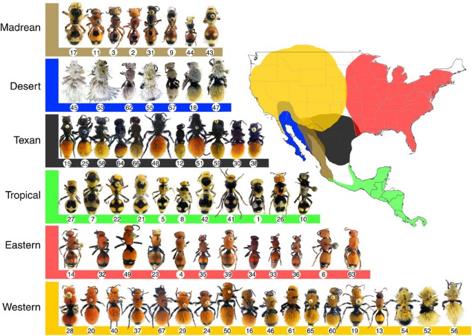Figure 1: Velvet ant mimicry rings. A total of 65Dasymutillaspecies (and three populations ofD. bioculata) are placed into six mimicry rings that are defined by shared colour, pattern and geographic location. Numbers under each species correspond to their position on the phylogenetic tree (Fig. 3) and toSupplementary Table S1, which contains voucher and collection locality information for each of the specimens used in the analyses. Figure 1: Velvet ant mimicry rings. A total of 65 Dasymutilla species (and three populations of D. bioculata ) are placed into six mimicry rings that are defined by shared colour, pattern and geographic location. Numbers under each species correspond to their position on the phylogenetic tree ( Fig. 3 ) and to Supplementary Table S1 , which contains voucher and collection locality information for each of the specimens used in the analyses. 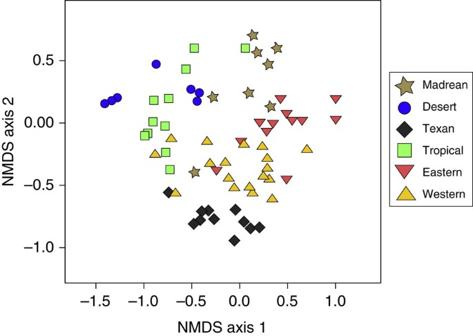Figure 2: Ordination plot of morphological characters. NMDS plot based on morphological characters from each of the six mimicry rings. Full size image Figure 2: Ordination plot of morphological characters. NMDS plot based on morphological characters from each of the six mimicry rings. Full size image Rather than naming each mimicry ring based on colour characteristics, as has often been done in butterfly mimicry rings [27] , we categorize each mimicry ring based on the geographic location of the ring (for example, Eastern, Western, Tropical, Desert, Texan and Madrean). The Madrean mimicry ring is named for the Sierra Madre Occidental Mountains and the Madrean Archipelago [28] , where it most commonly occurs. Species involved in the Madrean mimicry ring ( N =8) have reddish integumental colouration that is sharply marked with contrasting black, white, silver, gold or yellow setal and integumental patterns ( Fig. 1 ). Many of the species in this mimicry ring also have silver or golden setae on their head, and white or yellow markings on the second metasomal tergite (T2). Members of the Desert mimicry ring can be found primarily in the warm deserts of North America (Mojave, Sonoran, Peninsular and Chihuahuan) with most species concentrated in the Sonoran and Peninsular deserts. These species ( N =7) all share a common colour pattern of white setae on the head and mesosoma, with a white-to-pale yellow metasoma ( Fig. 1 ). Many species in this mimicry ring have black legs, petiole and venter, others are completely covered with white setae. The Texan mimicry ring can be found throughout Texas, southern New Mexico and northeastern Mexico. Members of this mimicry ring ( N =11) are characterized by having a black head and mesosoma with a reddish to orange metasoma ( Fig. 1 ). The Tropical mimicry ring can be found in the tropical regions of North America, from Panama through southern Mexico. Members of this mimicry ring ( N =11) share a pattern consisting of black integument with contrasting patterns of white or yellow setal markings ( Fig. 1 ). Frequently, there are yellow integumental spots on T2. The Eastern mimicry ring is found throughout eastern North America, with species ranging from the Atlantic coast to the central Great Plains. Members of this mimicry ring ( N =12) have orange-to-red integument with a sparse covering of setae on the head, mesosoma and the first several metasomal segments, but with contrasting patterns of silver, black or orange setae near the apex of the metasoma ( Fig. 1 ). The Western mimicry ring is found throughout western North America from the Pacific coast to the Great Plains. Members of this mimicry ring ( N =18) are all covered with dense, often shaggy yellow to red dorsal setae. Some species also have contrasting black setae on the legs, petiole and apex of the metasoma ( Fig. 1 ). Phylogenetic reconstructions To determine whether shared colour patterns could be attributed to phylogenetic history or if they are a result of repeated evolutionary events, we estimated phylogenetic relatedness using non-coding DNA markers (internal-transcribed spacer regions 1 and 2 (ITS1 and ITS2)), as well as a protein-coding marker (wingless). Both Bayesian phylogenetic analyses (using non-coding and protein-coding markers) resulted in phylogenies showing distinct colour forms spread across the genealogy with multiple colour forms present in well-supported clades ( Fig. 3 ). While the tree based on the protein-coding marker is less resolved than the tree based on the non-coding markers, the trees are largely concordant in the species that are placed into distinct, well-supported clades. Furthermore, the phylogenetic patterns found here are consistent with groupings based on structural morphological characters (that is, genitalic morphology) (K.A.W., unpublished data). Although no clear biogeographic signal is present among species, the general pattern is that of species inhabiting the Madrean Archipelago or tropical habitats generally having more ancient common ancestors relative to species inhabiting western North America. 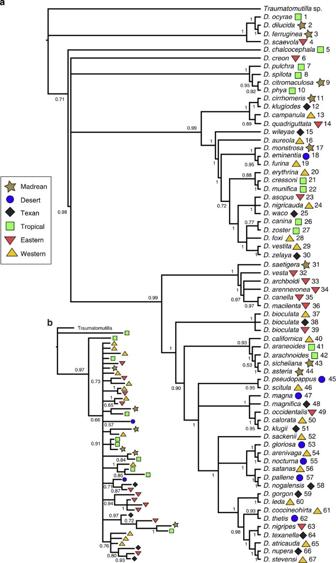Figure 3: Bayesian phylogenetic trees. Fifty per cent majority rules consensus trees based on neutral genetic loci (a) and protein-coding loci (b) with species coded with coloured circles representing the mimicry ring to which they belong (brown: Madrean; blue: Desert; black: Texan; green: Tropical; red: Eastern; yellow: Western). Numbers following each species correspond toFig. 1andSupplementary Table S1and can be used to associate the position of an individual species on the phylogeny to the image of that species inFig. 1. Posterior probabilities are given for each node. For ease of visualization, we have displayed the tree based on neutral genetic loci as ultrametric and the tree based on protein-coding loci as a phylogram. Figure 3: Bayesian phylogenetic trees. Fifty per cent majority rules consensus trees based on neutral genetic loci ( a ) and protein-coding loci ( b ) with species coded with coloured circles representing the mimicry ring to which they belong (brown: Madrean; blue: Desert; black: Texan; green: Tropical; red: Eastern; yellow: Western). Numbers following each species correspond to Fig. 1 and Supplementary Table S1 and can be used to associate the position of an individual species on the phylogeny to the image of that species in Fig. 1 . Posterior probabilities are given for each node. For ease of visualization, we have displayed the tree based on neutral genetic loci as ultrametric and the tree based on protein-coding loci as a phylogram. Full size image To establish whether shared colour patterns are randomly distributed on each phylogeny or if they might be attributed to phylogenetic relationships (that is, common descent), we compared our observed distribution of colour forms on each phylogeny to a null, random distribution. These analyses indicated that shared colour patterns in each mimicry ring are likely a result of repeated evolution and are not driven by phylogenetic relationships except possibly in the Eastern mimicry ring ( Table 1 ), where 5 of the 12 member species share a most recent common ancestor. Table 1 Results of Bayesian Tip-association significance testing for each mimicry ring. Full size table Müllerian mimicry rings have been described from a variety of North American taxa, including millipedes (seven species [6] ), eastern bumble bees (eight species [2] ) and the monarch and viceroy butterflies (two species [3] ), yet these mimetic systems often contain relatively few species. The butterfly genus Heliconius , which has become a model Müllerian system, contains 40 species, although other taxa are also involved with the Heliconius mimicry complexes. To our knowledge, the 65 Dasymutilla species treated here represent one of the largest Müllerian mimicry complexes yet to be identified, particularly in temperate regions. Although Heliconius mimicry rings have become the most widely known mimetic systems due to the variety of shared colour forms found in apparently distantly related species and populations [2] , [5] , recent analyses suggest that some phenotypes share a common origin within and between species [29] . These recent findings indicate that mimetic races within Heliconius species may be driven in part by shared phylogenetic history in addition to convergent evolution. Furthermore, analyses of recent genomic data sets have shown that a single mimetic phenotype can arise once and spread not only within species but also between species through hybridization, allowing multiple species to participate in the same mimicry rings [30] . Although genomic data and genetic data based on genes that code for colour are not available for velvet ants, future analyses might reveal similar patterns of hybridization or introgression among velvet ant species. While some amount of shared phylogenetic history is likely responsible for similarities in colour in some velvet ant species, most of the diversity in the Dasymutilla mimicry rings is at the level of species rather than races, with convergent coloration found even in distantly related species ( Figs 1 , 3 ). Divergence times for many of the species involved in mimicry rings are estimated to have started around 20 million years ago, with a majority of species arising between 10 and 5 million years ago [31] . A unique feature of this system is that mimicry within Dasymutilla rings is often achieved through convergence of different morphological features. For example, colour patterns can be based on setal colour and/or integumental pigmentation (for example, D. furina and D. campanula : Figs 1 , 3 ), supporting our finding of convergent evolution in colour pattern. In addition to mimicry among Dasymutilla species, other velvet ant taxa also share similar colour patterns with Dasymutilla . For example, members of the genus Pseudomethoca share colour patterns with members of each of the six mimicry rings described here. An additional eight velvet ant genera also appear to participate in the Tropical mimicry ring in Central America (K.A.W., personal observations). Several ecological characteristics make Dasymutilla unique among known mimetic complexes. Dasymutilla females, like all female velvet ants, are wingless. Velvet ants spend much of their adult lives searching for nests of their hosts in open soil or other exposed microhabitats. While birds are typically implicated as the predator driving the evolution of shared colour patterns in mimicry systems [7] , little evidence exists that birds regularly attack velvet ants. Instead, diurnal lizards have likely been the key selective agent in the evolution of Dasumutilla mimicry rings. Several North American lizard species regularly feed on insects with heavy exoskeletons and species armed with painful stings [11] . Feeding trials have shown that a velvet ant’s hard cuticle increased prey manipulation time for predators, often allowing the velvet ant to sting, which generally resulted in a release of the velvet ant with no significant damage [10] , [11] , [12] . These defenses, when combined with chemical, visual and auditory warning signals, separate velvet ant mimicry complexes from most other known mimicry systems because they are able to train potential predators without being consumed or mortally wounded. Furthermore, when a lizard predator is stung and releases a velvet ant, it is presented immediately with the velvet ant’s auditory and visual warnings. This combination of painful sting and aposematic signals encourages rapid learning, with many lizards completely avoiding a velvet ant after a single attempted predation event [11] . The ability of velvet ants to quickly train predators without sustaining injuries may have driven the rapid evolution of distinct colour forms in this group. While our analyses clearly delineate mimicry rings among female Dasymutilla species, several aspects of this mimicry complex remain unexplored and can potentially aid our understanding of aposematism and mimicry. Recent molecular analyses have found that several named velvet ant species actually comprise different colour forms of a single species [23] , [32] , [33] . Continued taxonomic investigations of Dasymutilla will certainly reveal more instances of multiple colour forms within a single species. While future taxonomic revisions can be expected, these are unlikely to change our findings of multiple origins of aposematic colouration. As shown in Fig. 3 , multiple geographically distributed colour forms are present in clades of closely related species (which future analyses may indicate are synonyms), but are also found across the phylogeny in very distantly related species. Although male velvet ants are relatively harmless compared with their female counterparts, they often exhibit aposematic colouration; these males could thus be Batesian mimics of female velvet ants. Interestingly, male velvet ants do not always match the same mimicry ring as their conspecific females. Sexual dimorphism also drives intraspecific colour variation, with winged males often bearing little resemblance to their conspecific females. Fewer than 30% of Dasymutilla species are known from both sexes (45 species known from both sexes; 127 known from only one sex). Continued use of molecular techniques to improve taxonomy [22] , [32] will reveal additional synonymies and sex associations, will facilitate studies of Batesian mimicry in male Dasymutilla and will undoubtedly add to our understanding of mimicry in this complex group. Yet another element of complexity in this system comes from the possibility that some of the colour patterns (that is, the Desert mimicry ring) might be cryptic rather than aposematic [10] , [21] . It is also possible that some colour syndromes are more effective aposematic signals than others. Velvet ants are kept easily in captivity, so the effectiveness of colour syndromes for training predators can be studied in laboratory settings. Also, while collections of Dasymutilla in the United States are fairly thorough, our knowledge of velvet ant diversity in Mexico remains incomplete. Additional investigations into velvet ant diversity in Mexico and Central America will likely add to our understanding of mimicry in velvet ants. Furthermore, additional putative mimicry rings exist in related velvet ant groups in South America and elsewhere. As additional collections are made and the necessary taxonomic work is completed, velvet ants can become a model system for studying aposematism and mimicry. Here we have documented a diverse mimicry complex among female Dasymutilla velvet ants and we have described six distinct mimicry rings (Eastern, Western, Tropical, Desert, Texan and Madrean). Morphometric analyses indicate that these mimicry rings are morphologically distinct. Phylogenetic analyses indicate that most of the similarity in colouration within mimicry rings is a result of repeated evolution rather than shared ancestry. To our knowledge, the Dasymutilla Müllerian mimicry rings represent one of the largest documented mimicry complexes both in terms of geographic area and species richness. The novel characteristics of the large Dasymutilla mimicry complex make them unique among known mimetic systems. Future studies of this group and other velvet ant complexes will likely add to our understanding of Müllerian and Batesian mimicry and could lead to velvet ants becoming model organisms for the study of the ecology and evolution of mimicry and aposematism. Sampling and study organism Specimens were collected from sites across North America from 2002 to 2011, primarily using malaise traps and by hand. All specimens were placed directly into 95% ethanol, and those used for molecular examination have been labelled as voucher specimens and deposited in the Department of Biology Insect Collection, Utah State University, Logan, Utah (EMUS). Morphological analyses We quantified seven colour characters and one setal character using digital images of each species ( Fig. 1 ) using ImageJ ( http://rsb.info.nih.gov/ij/ ). Colour characters were measured from digital images and included the per cent black of the mesosoma, per cent black of the metasoma, pattern on metasoma, integument colour and non-black metasomal colour measured in red, green and blue. Setal length was also recorded as a categorical variable with five possible categories. Morphological characters were analysed using NMDS based on a Bray–Curtis distance matrix and PERMANOVA [34] in R [35] using the adonis function in the vegan package. Following the discovery of an overall significant effect of ring in a PERMANOVA analysis on the complete data set, pairwise comparisons were conducted to investigate the distinctness of each pair of rings. Finally, we conducted a test (also with the vegan package) for homogeneity of dispersion, which is an assumption of the PERMANOVA approach (we did not detect significant differences in dispersion). Molecular and phylogenetic analyses Molecular methods, including DNA extraction, PCR, sequencing and alignment followed the protocols of Pilgrim and Pitts [22] and Pilgrim et al . [36] We amplified and sequenced a protein-coding marker, wingless, and two non-coding markers, ITS1 and ITS2. The non-coding and protein-coding markers were separately subjected to Bayesian analysis using MrBayes v3.1.2 (ref. 37 ). Neutral markers were analysed as a combined data set with each gene partitioned separately. The GTR+Γ model was applied to ITS1 and GTR+Γ+I applied to ITS2 as determined in MrModeltest version 2.3 (ref. 38 ). The protein-coding locus was analysed under the SYM+I+Γ model. Bayesian analyses included four independent runs with three heated chains and one cold chain in each run. The MCMC chains were set for 5,000,000 generations and sampled every 100 generations; chains were run until the average s.d. of the split frequencies dropped below 0.01. A 10% burn-in was removed after graphical determination of stationarity using Tracer v1.5 (ref. 39 ). A Traumatomutilla species was included as an outgroup. All sequences for each gene resulted in clean sequences, suggesting no gene heterogeneity and have been submitted to GenBank ( Supplementary Table S1 ). To establish whether shared colour patterns are randomly distributed on each phylogeny or if they might be attributed to phylogenetic relationships (that is, common descent), we used a Bayesian approach to compare our observed distribution of colour forms on each phylogeny with a null, random distribution using program BaTS (Bayesian Tip-association Significance testing [40] ). BaTS tests for significant phylogeny–trait correlations and accounts for phylogenetic uncertainty by integrating over the entire collection of post burn-in trees generated by the MrBayes analysis of each data set. We used 1,000 state randomizations to create the null distribution to test the significance of our observed data. Accession codes: The gene sequence data have been deposited in the GenBank nucleotide database under accession numbers DQ408497 , DQ408502 , EF433451 , EF433452 , EU367350 , EU627568 to EU627570 , EU627572 , HQ317244 to HQ317247 , HQ317254 , HQ317255 , HQ317257 , HQ317267 , HQ317268 , HQ317270 , HQ317276 , HQ317281 , HQ317288 , HQ317289 , JQ945768 to JQ945771 , JQ945773 , JQ945776 to JQ945786 , JQ945789 to JQ945792 , JQ945794 , JQ945797 to JQ945800 , JQ945802 to JQ945805 , JQ945807 , JQ945808 , JQ945811 , JQ945834 to JQ945837 , JQ945839 , JQ945843 to JQ945851 , JQ945858 to JQ945860 , JQ945862 , JQ945865 to JQ945869 , JQ945871 to JQ945874 , JQ945883 to JQ945885 , JQ945887 to JQ945890 , JQ945892 to JQ945896 , JQ945899 , JQ945909 to JQ945911 , JX002743 , JX002745 to JX002747 , JX002775 to JX002777 , JX002780 to JX002783 , JX002785 , JX002786 , JX002789 , JX002790 , JX002792 to JX002794 , JX002796 , JX002797 , JX002799 , JX002800 , JX002802 to JX002810 , JX002812 , JX002815 to JX002817 , JX002820 to JX002853 , JX002870 , JX002887 . How to cite this article: Wilson, J.S. et al . Repeated evolution in overlapping mimicry rings among North American velvet ants. Nat. Commun. 3:1272 doi: 10.1038/ncomms2275 (2012).